Metabolome-based genome-wide association study of maize kernel leads to novel biochemical insights Plants produce a variety of metabolites that have a critical role in growth and development. Here we present a comprehensive study of maize metabolism, combining genetic, metabolite and expression profiling methodologies to dissect the genetic basis of metabolic diversity in maize kernels. We quantify 983 metabolite features in 702 maize genotypes planted at multiple locations. We identify 1,459 significant locus–trait associations ( P ≤1.8 × 10 −6 ) across three environments through metabolite-based genome-wide association mapping. Most (58.5%) of the identified loci are supported by expression QTLs, and some (14.7%) are validated through linkage mapping. Re-sequencing and candidate gene association analysis identifies potential causal variants for five candidate genes involved in metabolic traits. Two of these genes were further validated by mutant and transgenic analysis. Metabolite features associated with kernel weight could be used as biomarkers to facilitate genetic improvement of maize. Plants produce numerous structurally diverse metabolites, which play essential roles in growth, cellular replenishment and whole-plant resource allocation as well as roles in plant development and stress responses. In addition, they provide essential resources for human nutrition, bioenergy, medicine, flavourings, and so on [1] . Understanding plant biochemistry is thus of fundamental importance for sustainable agriculture and resource conservation, especially under changing climate conditions [2] . Metabolomics, which enables comprehensive high-throughput quantification of a broad range of metabolites, is invaluable for both phenotyping and diagnostic studies in humans, animals and plants [3] , [4] , [5] . The importance of maize as one of the critical crops for food and feed worldwide makes a comprehensive metabolomic study of this species imperative [6] , [7] , [8] . Moreover, maize manifests exceptional genome and phenotypic diversity among its inbred lines [9] , [10] , making it an attractive model organism for crop genetics. As the perceived end product of cellular regulatory and metabolic processes, the metabolite spectrum and quantities making up the metabolic complement may be viewed as the metabolic phenotype or metabotype [11] , [12] . As the metabolic phenotype provides a link between gene sequence and visible phenotypes, metabolites can be used as biomarkers for trait prediction [6] , [13] . In humans, genome-wide association studies (GWAS) are beginning to unravel the genetics of metabolic traits and demonstrate their utility in biomedical and pharmaceutical research [14] . Numerous studies on plant primary and secondary metabolites have been carried out that allowed the detection of hundreds of QTLs in Arabidopsis, rice and tomato [15] , [16] , [17] , [18] . Recently, the first metabolite-based association study in maize demonstrated the utility of this approach in genetic improvement [7] . However, the understanding of the genetic and molecular basis of natural variation in plant metabolomes, including those of maize, is still limited to relatively small population size and a few selected biochemical pathways [7] , [15] , [16] , [17] , [18] . Further, despite of the respective advantages of GWAS, it is logical to borrow the strengths from linkage analysis to complement GWAS in order to validate and identify causal polymorphisms [19] . The rapid development of RNA sequencing and metabolomic technologies coupled with SNP data has enabled eQTL and mQTL mapping at a large scale that help us to understand the flow of biology information underlying complex traits in the systems genetics level [20] . Combing GWAS and transcript data can allow the rapid identification of a large number of novel genes and potential networks that affect specific metabolism, as suggested by a previous study in Arabidopsis thaliana [21] . Recently, we obtained expression data of 28,769 genes and ~1 million high-quality SNPs by deep RNA sequencing of the immature seeds of 368 diverse maize inbreds [22] . A pilot GWAS for oil concentration and composition in maize kernels has identified 74 loci associated with target traits that explain the majority of the observed phenotypic variation [23] . Here we analyse 184 metabolites with associated chemical structures and additional 799 unknown metabolite features, using 368 diverse maize inbreds, SNP and gene expression information as mentioned above, along with two recombinant inbred (RIL) populations. We reveal a relatively simple genetic architecture for most metabotype compositions using GWAS and linkage mapping analysis. GWAS manifests strong power to dissect metabolite traits and its findings can be validated using linkage and eQTL analysis, as well as functional validation through molecular experiments. We find novel metabolites and genes, constituting key processes in the formation of phenolamides (PAs) and flavonoids. Combining genetics, metabolomics and expression profiles significantly improves our knowledge of both the functional genomics and metabolism of maize and provides a powerful tool for crop improvement. Metabolite profiling Using high-throughput LC-MS/MS analysis, we detected and quantified 983 distinct metabolite features from mature kernel extracts of the association panel (368 inbred lines) harvested at three locations in China. Most of them (793/983) were also detected in the two RIL populations (334 lines), as well as overlapped metabolite features found in replications of the association panel ( Supplementary Fig. 1 ). Chemical structures of 184 metabolites were identified or annotated ( Supplementary Data 1 and 2 ). The level of each metabolite feature varied widely across the lines in both the association panel and linkage populations. For the intensity of a majority of metabolite features (>83% in the association panel, >66% in the linkage population), >10-fold change difference measured in each experiment was observed ( Supplementary Fig. 2 ), indicating high natural variability. Greater phenotypic diversity for these metabolite features was observed among the lines of the association panel than within both linkage populations ( Supplementary Fig. 2 ). In the association panel, 725 metabolite features were detected in two or three environments, 71.7% of which were observed with a repeatability of >0.5, and 48.3% with a repeatability of >0.7 ( Supplementary Fig. 3 ). The level of repeatability indicated a precise phenotyping of metabolic level measurement and a significant genetic contribution to the determination of metabolic content within the association panel and the three experiments. GWAS was performed for each experiment independently as the level of replication within each experiment was not sufficient to directly test the genotype by experiment interaction term. Genetic basis of maize metabolome In GWAS, >45% of the metabolite features in each of the three environments had at least one associated locus at a genome-wide significance level of P ≤1.8 × 10 −6 (calculated by mixed linear model controlling Q and K (MLM); N =335–339). 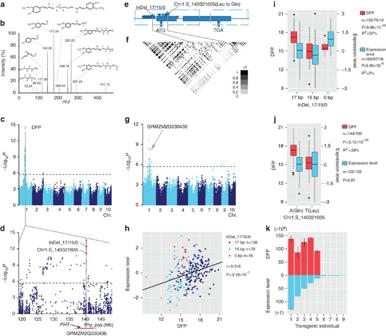Figure 1: Casual sites identification and functional validation of putrescinehydroxycinnamoyltransferase. (a) Structure ofN,N-Di-feruloylputrescine (DFP or DiFer-Put) in the polyamine pathway. (b) LC/MS fragmentation of DFP. Possible structures of the major fragments are shown. (c) Manhattan plot displaying the GWAS result of the content of DFP (MLM,N=339). (d) Regional association plot for locusPHT. The significant sites identified by re-sequencingPHT(GRMZM2G030436), show in red (MLM,N=230~320). The bigger red points show the putative functional polymorphisms, an insertion/deletion at the site InDel_17/15/0 and a SNP at Chr1.S_140321605. (e) Gene model ofPHT. Filled blue boxes represent exons and UTRs. The dashed boxes mark the re-sequenced region, and the stars represent the significant sites identified by re-sequencing, the bigger stars represent the proposed functional sites. (f) A representation of the pair-wiser2value among all polymorphic sites inPHT, where the colour of each box corresponds to ther2value according to the legend. (g) Manhattan plot shows the association between expression level ofPHTand genome-wide SNPs. Significant signals are mapped to SNPs withinPHT, indicating acistranscriptional regulation of this gene (MLM,N=368). The presence of the proposed functional site, InDel_17/15/0, is associated with both the expression level and the content of DFP (h,i), implying that the changed expression level is partially responsible for the change in DFP content. (h) Plot of correlation between the content of DFP and the normalized expression level of thePHTgene. Maize inbred lines with different genotypes at the InDel_17/15/0 site were shown in red, sky blue and midnight blue, respectively. Thervalue is based on a Pearson correlation coefficient. ThePvalue is calculated using thetapproximation. (i) Box plot for DFP content (red) and expression ofPHT(sky blue); plotted as a function of genotypes at the site InDel_17/15/0. (j) Box plot for DFP content (red) and expression ofPHT(sky blue), plotted as a function of genotypes at the site Chr1.S_140321605. Horizontal line represents the mean and vertical lines mark the range from 5th and 95th percentile of the total data (i,j), respectively. (k) Bar plot for DFP content andPHTexpression level in rice transgenic individuals (T0). The content of DFP and expression level ofPHTin the leaves of each transgenic individual is shown in red and sky blue, respectively. Vertical lines represent the s.e. (N=3). In total, 1,459 distinct locus–trait associations were identified across three environments ( Table 1 ; Supplementary Data 3 ). Each locus explained 5.7–49.1% of the observed metabolic variance, with a median of 7.8%. Among 725 metabolite features that were detected in more than one environment, we found a total of 1,256 significant loci associated with 501 of them ( P ≤1.8 × 10 −6 ). Of the 1,256 associations, 210 (16.7%) were consistently identified in two or three environments at P ≤1.8 × 10 −6 ( Supplementary Data 3 ). Additionally, with relaxed cutoff values of P ≤1.8 × 10 −6 in one environment and P ≤1.0 × 10 −4 in at least one of the other two environments, the proportion of significant locus–trait associations that are found in at least two environments increased to 50.2% ( Supplementary Data 3 ). Table 1 Summary of significant loci–trait associations identified by GWAS and QTL identified by linkage mapping. Full size table Linkage mapping in the BB RIL population identified 1,152 QTLs for 550 metabolite features, which accounted for 75.9% of all metabolic traits detected in this population. For the ZY RIL population, 60.7% traits (447 of 736) had at least one QTL ( Table 1 ). Each QTL explained 3.3–80.4% (in the BB RIL) and 5.3–65.6% (in the ZY RIL) of the phenotypic variance ( Supplementary Data 4 ). Of the significant GWAS loci identified in three environments, 14.7% overlapped with the QTLs identified in at least one of the two RIL populations ( Supplementary Data 3 and 4 ). In the present study, 1,197 unique candidate genes corresponding to 1,459 significant locus–trait associations identified across three environments were annotated ( Supplementary Data 3 ; only the nearest candidate was reported here, but for the metabolites with identified or annotated structure, genes within a 100-kb flanking region of the lead SNPs were also provided in Supplementary Data 5 ). Cis expression QTLs (eQTL, P ≤1.8 × 10 −6 , MLM, N =368) were identified for the majority of these candidate genes (58.5% or 700/1,197), which were from 946 significant locus–trait associations identified across three environments. Within these 946 locus–trait associations, significant correlation ( P ≤0.01, t approximation, N =335–339) between the expression level of the candidate genes and the phenotypic variation of the target metabolic traits were found in 238 cases (25.2%), which implied that at least some of these candidate genes affect the phenotypic variation via transcriptional regulation. Functions of 24% of these genes are currently unknown based on the available database. Catalytic enzymes, regulators and transporters were involved in the metabolite content control ( Supplementary Fig. 4 ). Biochemical and functional interpretation of GWAS results The utility of a metabolic phenotype is enhanced by the rich knowledge base of many metabolic pathways and the ability to corroborate candidate associations with biological and functional arguments [12] , [24] . In addition, using GWAS on these metabolic phenotypes, we were able to verify and have the chance to update the annotation of many maize genes. Correlating gene annotation and the biochemical characteristics of the associated metabolite frequently allows selection of a single most likely causative gene. 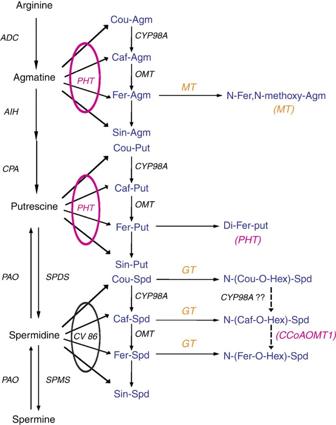Figure 2: Proposed pathway of polyamine conjugates biosynthesis. The common conjugates are indicated in blue and new candidate genes in red (confirmed) and golden (not verified). ADC, arginine decarboxylase; AIH, agmatineiminohydrolase; CPA,N-carbamoylputrescineamidohydrolase; DAO, diamine oxidase; SPDS, spermidinesynthase; SPMS, spermine synthase; PAO, polyamine oxidase; PHT, putrescine: hydroxycinnamoyltransferase; GT, glycosyltransferase; CCoAOMT1, caffeoyl-CoAO- methyltransferase 1. Candidate gene revealed by the association analysis was put in the bracket under the corresponding metabolite. The association between caffeoyl CoA 3- O -methyltransferase 1( CCoAOMT1 ) [25] , [26] and caffeic acid, dicaffeoylspermidine and several other metabolites is one example of easily pinpointing the most likely causative gene ( Table 2 and Supplementary Data 3 ). GWAS associations with N , N -Di-feruloylputrescine and Apigenin di- C -pentoside provided us the opportunity to potentially update functional annotation of their causal genes ( Fig. 1 ; Table 2 and Supplementary Data 3 ). On the other hand, the annotation of candidate genes provides useful clues to the biochemical nature of the associated metabolites. Locus TDC1 (tryptophan decarboxylase, located on chromosome 10 at 82851072bp), which was significantly associated with 16 metabolites ( P =7.21 × 10 −18 –1.54 × 10 −6 , MLM, N =335–339), contains two highly homologous genes (GRMZM2G021277 and GRMZM2G021388, 89% and 88% DNA and amino-acid homology, respectively). Their annotated function in Hordeumvulgare is tryptophan decarboxylase (IPR010977, query coverage 99% and max identity 86%).We predicted that some of these 16 metabolites are tryptophan derivatives based on tryptamine (3-(2-Aminoethyl) indole hydrochloride) standard ( Table 2 and Supplementary Data 3 ). Likewise, GWAS result of metabolite n0769 and functional annotation of the candidate gene (steroleosin, STE ) suggested the structure of n0769 ( Table 2 and Supplementary Data 3 ). STE is a sterol-binding dehydrogenase in seed oil bodies [27] . Indeed, n0769 could be fatty acid moiety—suggested by its mass spectrum fragmentation pattern, even though the complete structure remains to be determined. Table 2 Validation of candidate genes through various methodologies and associated information. Full size table Figure 1: Casual sites identification and functional validation of putrescinehydroxycinnamoyltransferase. ( a ) Structure of N , N -Di-feruloylputrescine (DFP or DiFer-Put) in the polyamine pathway. ( b ) LC/MS fragmentation of DFP. Possible structures of the major fragments are shown. ( c ) Manhattan plot displaying the GWAS result of the content of DFP (MLM, N =339). ( d ) Regional association plot for locus PHT . The significant sites identified by re-sequencing PHT (GRMZM2G030436), show in red (MLM, N =230~320). The bigger red points show the putative functional polymorphisms, an insertion/deletion at the site InDel_17/15/0 and a SNP at Chr1.S_140321605. ( e ) Gene model of PHT . Filled blue boxes represent exons and UTRs. The dashed boxes mark the re-sequenced region, and the stars represent the significant sites identified by re-sequencing, the bigger stars represent the proposed functional sites. ( f ) A representation of the pair-wise r 2 value among all polymorphic sites in PHT , where the colour of each box corresponds to the r 2 value according to the legend. ( g ) Manhattan plot shows the association between expression level of PHT and genome-wide SNPs. Significant signals are mapped to SNPs within PHT , indicating a cis transcriptional regulation of this gene (MLM, N =368). The presence of the proposed functional site, InDel_17/15/0, is associated with both the expression level and the content of DFP ( h , i ), implying that the changed expression level is partially responsible for the change in DFP content. ( h ) Plot of correlation between the content of DFP and the normalized expression level of the PHT gene. Maize inbred lines with different genotypes at the InDel_17/15/0 site were shown in red, sky blue and midnight blue, respectively. The r value is based on a Pearson correlation coefficient. The P value is calculated using the t approximation. ( i ) Box plot for DFP content (red) and expression of PHT (sky blue); plotted as a function of genotypes at the site InDel_17/15/0. ( j ) Box plot for DFP content (red) and expression of PHT (sky blue), plotted as a function of genotypes at the site Chr1.S_140321605. Horizontal line represents the mean and vertical lines mark the range from 5th and 95th percentile of the total data ( i , j ), respectively. ( k ) Bar plot for DFP content and PHT expression level in rice transgenic individuals (T0). The content of DFP and expression level of PHT in the leaves of each transgenic individual is shown in red and sky blue, respectively. Vertical lines represent the s.e. ( N =3). Full size image Functional validation of candidate genes To further validate GWAS findings and investigate functional variations in the candidate sequences, we tested five representative genes, PHT (putrescinehydroxycinnamoyltransferase), CCoAOMT1 , STE , UGT (UDP glycosyltransferase) and TDC1 , using multiple molecular approaches. These included re-sequencing PCR products that encompassed the genetically associated polymorphisms in the relevant inbred lines, eQTL analysis, linkage analysis, mutant analysis and/or transgenic expression. The PHT locus (GRMZM2G030436) showed the highest significance ( P =2.57 × 10 −15 , MLM, N =339, Supplementary Data 3 ) in the association with the content of compound N , N -Di-feruloylputrescine (DFP) in maize [28] . We further verified its function by transgenic analysis in rice ( Table 2 and Fig. 1 ). Over-expression of PHT in rice resulted in the accumulation of DFP in the leaf tissue in which it is normally absent, which strongly suggest the involvement of PHT in the biosynthesis of DFP ( Supplementary Fig. 5 ). The functional annotation of PHT was thus updated from transferase (IPR003480) to a putative putrescinehydroxycinnamoyltransferase. Re-sequencing uncovered a 0/15/17bp InDel polymorphism in the promoter region, which is the most likely responsible for the natural variation of DFP content, as well as the expression difference of PHT . Re-sequencing also identified five polymorphisms in the first exon that were significantly associated with the target traits ( P =4.34 × 10 −14 –1.26 × 10 −11 , MLM, N =230–320) and in modest-to-high LD with the InDel identified in the promoter region ( r 2 =0.48–0.81). One of the polymorphisms caused the deletion of an amino acid, and three resulted in amino-acid replacements ( Supplementary Table 1 and 2 ). Taken together, genetic variants within promoter and exon regions might contribute to the functional variation of PHT ( Fig. 1 ). CCoAOMT1 (GRMZM2G127948) encodes a Caffeoyl-CoA O -methyltransferase. It influences the content of several metabolites, and its function was validated by examining both CCoAOMT1 knockout maize lines and transgenic rice lines ( Table 2 and Supplementary Fig. 6 ). A monoacylatedagmatine, putrescine and an unknown spermidine derivative (S11) were significantly upregulated in the CCoAOMT1 knockout lines ( Supplementary Fig. 5 ). The association between its allelic variations and the metabolite n1544-1 (spermidine derivative S11) was supported by metabolite QTL mapping in both BB and ZY RIL populations. After re-sequencing the association panel, a strong association signal was detected with a 28 bp InDel in the 5′ untranslated region (UTR) of CCoAOMT1 ( P =1.99 × 10 −22 , MLM, N =315, Supplementary Table 1 and 2 and Supplementary Fig. 6 ). At the site of this InDel, the parents of the ZY RIL population, but not of the BB RIL population are polymorphic, suggesting that the 28-bp InDel might not be causative, or not the only causative sequence change. The negative correlation between metabolite content and gene expression level suggested that transcriptional regulation may cause the phenotype, although the 28-bp InDel is only marginally correlated ( P =0.06, t approximation, N =315) with gene expression ( Supplementary Table 1 and Supplementary Fig. 6 ). In STE (GRMZM2G108338), re-sequencing revealed a 1-bp InDel in the coding region, causing a frame shift that was significantly associated with the content of n0769 ( P =3.8 × 10 −8 , MLM, N =326, Supplementary Table 1 and 2 and Supplementary Fig. 7 ). We also found a significant difference between the expression levels of the two alleles at this InDel ( P =0.02, t -test, N =326, Supplementary Fig. 7 ). In addition, a strong cis eQTL was detected for STE ( P =1.4 × 10 −18 , MLM, N =368, Supplementary Fig. 7 ), and the expression level of this gene was positively correlated with the quantity of n0769 measured ( r =0.21, P =7.8 × 10 −4 , N =339; Table 2 and Supplementary Fig. 7 ). Re-sequencing the promoter region of STE indicated that another potentially causative polymorphism (an 878/185 bp InDel located 370 bp upstream of STE ) was strongly associated with the STE expression level ( P =3.7 × 10 −13 , ANOVA, N =263, Supplementary Table 1 and Supplementary Fig. 7 ) and slightly associated with the phenotypic trait ( P =0.003, AVONA, N =263, Supplementary Fig. 7 ). Low LD ( r 2 =0.02) was observed between the two polymorphisms. We thus postulate that the two InDels are both associated with phenotypic and expression variation to different extents. UGT (GRMZM2G383404), annotated as UDP-glycosyltransferase, was associated with the natural variation of a flavonoid putatively named Apigenin di- C -pentoside. Despite the fact that it is homologous to rice gene anthocyanin-3- O -glycosyltransferase, the protein sequence similarity of UGT to rice flavone-6- C -glucosyltransferase (Os06g18010) is higher than the anthocyanin-3- O -glucosyltransferase gene in maize (also known as Bz1 GRMZM2G165390; Supplementary Fig. 8 ) [29] , [30] . Strongly associated SNPs were identified in UGT by re-sequencing ( Supplementary Table 1 and 2 ). Eight significant SNPs found in the exon region were located in a LD block. Six of these eight SNPs cause substitution of amino acids and one SNP (A/C, SYN13426; P =1.1 × 10 −9 , MLM, N =316) results in amino-acid polarity change (Asp to Ala). This and other SNPs in the LD block are likely to constitute the functional variation; however, it is difficult to exclude other variants surrounding this region ( Supplementary Table 1 and Supplementary Fig. 9 ). A 602-bp InDel in the promoter region of TDC1 (GRMZM2G021277), identified by re-sequencing, is significantly associated with tryptamine content ( P =4.8 × 10 −14 , MLM, N =309; Supplementary Table 2 ). TDC1 was located within the QTL region mapped in the ZY RIL population and the 602-bp InDel was segregating in the parents. Although expression level of this gene in 60 tissues in maize is extremely low [31] and was not detected in our RNA-sequencing study [22] , this large InDel may affect the gene expression and, consequently, the phenotype ( Supplementary Table 1 and Supplementary Fig. 10 ). New genes in phenolamide and flavonoid biosynthesis pathways PAs, which are frequently referred to as hydroxycinnamic acid amides and phenylamides, have been identified in many plant species. PAs participate in many physiological and developmental processes [32] , [33] , [34] , related to defence against abiotic (temperature, drought and salt, and UV) and biotic (pathogen and insects) [33] , [34] , [35] , [36] , [37] stresses in plants. One of the major secondary metabolite groups in plants, flavonoids, is widely distributed and has a variety of functions [38] . Combining metabolomics analysis and GWAS, we found novel metabolites and genes constituting key processes in the formation of PAs and flavonoids, which had not been previously characterized in maize. In the biosynthesis of phenolamides, N -hydrocinnamoyltransferasesthatuse aliphatic amines as acyl acceptors and hydroxycinnamoyl-CoA as a donor were considered the key enzymes. Some were identified in plants, such as ACT (Agmatinecoumaroyltransferase) in barley [39] , SDT (spermidinesinapoyl CoA acyltransferase) and SCT (spermidinecoumaroyl CoA acyltransferase) in Arabidopsis [32] and AT1 (acyltransferase1), DH29 (acyltransferase DH29) and CV86 (acyltransferase CV86) in tobacco [40] . In addition, the conjugates can be further modified via species-specific hydroxylation, methylation, cyclization and coupling reactions [41] . In Arabidopsis , AtTSM1 , which encodes a CCoAOMT -like protein, was proven to have methylation activity in the biosysnthesis of phenolamides [42] . In this study, we quantified 27 phenolamides. GWAS indicated that locus PHT (GRMZM2G030436) was highly associated with the metabolite diferuloylputrescine (P6), while CCoAOMT1 (GRMZM2G127948) was responsible for the content of N -(caffeoyl- O -hexoside)-spermidine (S8) and two of N , N -caffeoyl,feruloyl-spermidine derivatives (S10 and 11) ( Supplementary Data 3 and Supplementary Fig. 5 ). PHT has 38% amino acid identity with previously identified AT1 from Nicotianaattenuata [40] and CCoAOMT 1 shows 81% identity with CCoAOMT1 from Arabidopsis thaliana [42] . The in vivo function of PHT and CCoAOMT1 were validated in this study as described above. In the rice PHT over-expression lines, both agmatine- and putrescine-associated conjugates were significantly upregulated ( Supplementary Fig. 5 ). Interestingly, no change of the monoacylated spermidine was observed while some of the diacylated spermidines were downregulated in the PHT -over-expressing lines ( Supplementary Fig. 5 ). In addition, some monoacylated agmatine and putrescine were significantly upregulated in the CCoAOMT1 knockout lines ( Supplementary Fig. 5 ), which further confirmed its biochemical function in vivo . Unlike the agmatineacyl transferase ( ACT ) [39] and putrescineacyltransferase ( AT 1) [40] reported previously, the PHT in our study seems to have a broader substrate specificity and can recognize both agmatine and putrescine, which has similar function with AtACT in Arabidopsis thaliana [43] . The lack of hydroxycinnamoyl-CoA may result in the downregulation of diacylatedspermidine in PHT- overexpressing lines. Therefore, we conclude that the PHT is likely an acyltransferase that can act on both agmatine and putrescine in maize. Furthermore, the latter modification of PAs in maize was also confirmed in CCoAOMT1 knockout lines ( Supplementary Fig. 5 ). Further, based on the results inferred by the metabolic profiling of our over-expressing rice lines and knockout maize lines, the biosynthetic pathway of phenolamides was reconstructed ( Fig. 2 ). Figure 2: Proposed pathway of polyamine conjugates biosynthesis. The common conjugates are indicated in blue and new candidate genes in red (confirmed) and golden (not verified). ADC, arginine decarboxylase; AIH, agmatineiminohydrolase; CPA, N -carbamoylputrescineamidohydrolase; DAO, diamine oxidase; SPDS, spermidinesynthase; SPMS, spermine synthase; PAO, polyamine oxidase; PHT, putrescine: hydroxycinnamoyltransferase; GT, glycosyltransferase; CCoAOMT1, caffeoyl-CoA O - methyltransferase 1. Candidate gene revealed by the association analysis was put in the bracket under the corresponding metabolite. Full size image Flavonol derivatives are highly enriched in mature maize kernels; flavanone and anthocyanin derivatives were also identified in our study. Based on the natural variation of these compounds, genomic loci responsible for the abundance of these flavonoids were identified ( Fig. 3 ). Genes involved in the regulation, as well as the biosynthesis, of individual steps in the flavonoid biosynthetic pathways were among these loci ( Fig. 3 and Supplementary Data 3 ). Notably, a known locus P1 , which encodes a R2R3-MYB transcription factor [44] , was responsible for natural variation of 20 flavonoids found in this study ( Supplementary Data 3 ). More interestingly, a considerable number of loci identified in this study as associated with flavonoids were direct targets of (or regulated by) P1 , as illustrated by Morohashi et al. [45] Functional annotation of these loci, including ABCT (ABC transporter; GRMZM2G018074), GRD2 (Glucose/ribitol dehydrogenase; GRMZM2G170013), HCT (hydroxycinnamoyl-CoA shikimate/quinatehydroxycinnamoyltransferase; GRMZM2G156816), UGT (UDP-glycosyltransferase; GRMZM2G383404), HLY (hemolysin-III homologue; GRMZM2G114650), UGT88A1 (UDP-glycosyltransferase 88A1; GRMZM2G122072) and SAMDC ( S -adenosylmethionine decarboxylase proenzyme Precursor; GRMZM2G154397), provided important clues for their involvement in maize flavonoid biosynthesis ( Fig. 3 ). Further experimental investigations are needed to elucidate the precise functions of these loci. 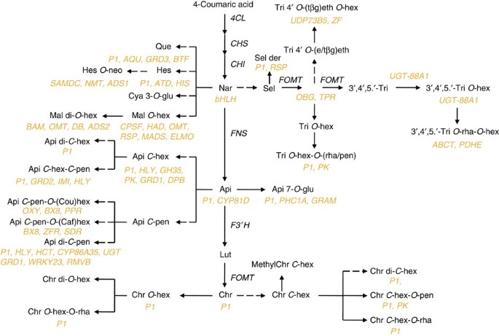Figure 3: Proposed pathway of flavonoid biosynthesis in maize kernel. Candidate genes identified by GWAS are shown in orange, under the corresponding associated metabolites. Api, Apigenin; Chr, chrysoeriol; Lut, Luteolin; cafpen, caffeoylpentoside; couhex, coumaroylhexoside; Cya, Cyanidin; der, derivative; glc, glucose; hes, hesperetin; hex, hexose; MethylChr, Methylchrysoeriol; Mal, Malvidin; pen, pentose; rha, rhamnose; Sel, Selgin; Tri, trincin; 3′,4′,5′-Tri, 3′,4′,5′-tricetin,(eβg)eth, (erythro-β-guaiacylglyceryl)ether; (tβg)eth, (threo-β-guaiacylglyceryl)ether; 4CL, 4-coumarate-CoA ligase; CHS, chalcone synthase; CHI, chalconeisomerase; FNS, flavone synthase; F3’H, flavonoid 3'-hydroxylase; FOMT, flavonoid O-methyltransferase; bHLH, basic helix-loop-helix (GRMZM2G162382); CPSF, cleavage and polyadenylation specificity factor 73-I(GRMZM2G422649); HAD, haloaciddehalogenase-like hydrolase superfamily(GRMZM2G035651); OMT,O-methyltransferase (GRMZM2G104710); RSP, ribosomal protein (GRMZM2G344279); MADS, MADS-box family protein (GRMZM2G129034); ELMO, ELMO/CED-12 family protein (GRMZM2G031952); BAM, beta-amylase (GRMZM2G069486); DB, DNA-binding (GRMZM2G478370); ADS, AMP-dependent synthetase and ligase (GRMZM2G019746); IMI, plant invertase/pectin methylesterase inhibitor superfamily (GRMZM2G054225); P1, MYB R2R3type transcription factor (GRMZM2G084799); AQU, aquaporin NIP-type (GRMZM2G126582); GRD2, glucose/ribitol dehydrogenase (GRMZM2G170013); GRD3, glucose/ribitol dehydrogenase (GRMZM2G059361); BTF, basic transcription factor(GRMZM2G110116); ATD, acetamidase/formamidasefamily protein (GRMZM2G424857); HIS, histone superfamily protein (GRMZM2G176358); UGT88A1, UDP-glycosyltransferase 88A1 (GRMZM2G122072); ABCT, ABC transporter (GRMZM2G018074); PDHE, erythronate-4-phosphate dehydrogenase family protein (GRMZM2G177982); RSP, 60S ribosomal protein (GRMZM2G344279); OBG, GTP1/OBG family protein (GRMZM2G077632); TPR, tetratricopeptide repeat (TPR)-like superfamily protein (GRMZM2G177072); SDH, succinate dehydrogenase (GRMZM2G134134); ABCB2, ABC transporter group B2 (GRMZM2G156145); PK, pyruvate kinase (GRMZM2G119175); UGT73B5: UDP-glycosyltransferase 73B5 (GRMZM5G888620); ZF, RING/U-box superfamily protein zinc finger (GRMZM2G145104); SAMDC,S-adenosylmethionine decarboxylase proenzyme Precursor (GRMZM2G154397); NMT, histone-lysineN-methyltransferase (GRMZM2G025924); RHC1A, RING-H2 finger C1A (GRMZM2G176028); GRAM, GRAM domain family protein (GRMZM2G106622); HLY, hemolysin-III homologue (GRMZM2G114650);GH35, glycoside hydrolase, family 35 (GRMZM2G153200); GRD1, glucose/ribitol dehydrogenase (GRMZM2G076981); DPB, DNA binding and protein binding (GRMZM2G393471); HCT, hydroxycinnamoyl-CoA shikimate/quinatehydroxycinnamoyltransferase (GRMZM2G156816); CYP86A35, cytochrome P450 family 86, subfamily A, polypeptide 35 (GRMZM2G062151); UGT, UDP glycosyltransferases (GRMZM2G383404); WRKY53, superfamily of transcriptional factors having WRKY and zinc finger domains (GRMZM2G449681); RMVB, regulator of Vps4 activity in the MVB pathway protein (GRMZM2G059590); bx8, benzoxazinone synthesis 8 (GRMZM2G085054); ZFR, zinc finger, RING-CH-type (GRMZM2G358987); SDR, short-chain dehydrogenase/reductase (GRMZM2G000586); OXY, 2OG-Fe(II) oxygenase superfamily (GRMZM5G843555); PPR, PPR repeat domain containing protein (GRMZM2G325019). Figure 3: Proposed pathway of flavonoid biosynthesis in maize kernel. Candidate genes identified by GWAS are shown in orange, under the corresponding associated metabolites. Api, Apigenin; Chr, chrysoeriol; Lut, Luteolin; cafpen, caffeoylpentoside; couhex, coumaroylhexoside; Cya, Cyanidin; der, derivative; glc, glucose; hes, hesperetin; hex, hexose; MethylChr, Methylchrysoeriol; Mal, Malvidin; pen, pentose; rha, rhamnose; Sel, Selgin; Tri, trincin; 3′,4′,5′-Tri, 3′,4′,5′-tricetin,(eβg)eth, (erythro-β-guaiacylglyceryl)ether; (tβg)eth, (threo-β-guaiacylglyceryl)ether; 4CL, 4-coumarate-CoA ligase; CHS, chalcone synthase; CHI, chalconeisomerase; FNS, flavone synthase; F3’H, flavonoid 3'-hydroxylase; FOMT, flavonoid O-methyltransferase; bHLH, basic helix-loop-helix (GRMZM2G162382); CPSF, cleavage and polyadenylation specificity factor 73-I(GRMZM2G422649); HAD, haloaciddehalogenase-like hydrolase superfamily(GRMZM2G035651); OMT, O -methyltransferase (GRMZM2G104710); RSP, ribosomal protein (GRMZM2G344279); MADS, MADS-box family protein (GRMZM2G129034); ELMO, ELMO/CED-12 family protein (GRMZM2G031952); BAM, beta-amylase (GRMZM2G069486); DB, DNA-binding (GRMZM2G478370); ADS, AMP-dependent synthetase and ligase (GRMZM2G019746); IMI, plant invertase/pectin methylesterase inhibitor superfamily (GRMZM2G054225); P1, MYB R2R3type transcription factor (GRMZM2G084799); AQU, aquaporin NIP-type (GRMZM2G126582); GRD2, glucose/ribitol dehydrogenase (GRMZM2G170013); GRD3, glucose/ribitol dehydrogenase (GRMZM2G059361); BTF, basic transcription factor(GRMZM2G110116); ATD, acetamidase/formamidasefamily protein (GRMZM2G424857); HIS, histone superfamily protein (GRMZM2G176358); UGT88A1, UDP-glycosyltransferase 88A1 (GRMZM2G122072); ABCT, ABC transporter (GRMZM2G018074); PDHE, erythronate-4-phosphate dehydrogenase family protein (GRMZM2G177982); RSP, 60S ribosomal protein (GRMZM2G344279); OBG, GTP1/OBG family protein (GRMZM2G077632); TPR, tetratricopeptide repeat (TPR)-like superfamily protein (GRMZM2G177072); SDH, succinate dehydrogenase (GRMZM2G134134); ABCB2, ABC transporter group B2 (GRMZM2G156145); PK, pyruvate kinase (GRMZM2G119175); UGT73B5: UDP-glycosyltransferase 73B5 (GRMZM5G888620); ZF, RING/U-box superfamily protein zinc finger (GRMZM2G145104); SAMDC, S -adenosylmethionine decarboxylase proenzyme Precursor (GRMZM2G154397); NMT, histone-lysine N -methyltransferase (GRMZM2G025924); RHC1A, RING-H2 finger C1A (GRMZM2G176028); GRAM, GRAM domain family protein (GRMZM2G106622); HLY, hemolysin-III homologue (GRMZM2G114650);GH35, glycoside hydrolase, family 35 (GRMZM2G153200); GRD1, glucose/ribitol dehydrogenase (GRMZM2G076981); DPB, DNA binding and protein binding (GRMZM2G393471); HCT, hydroxycinnamoyl-CoA shikimate/quinatehydroxycinnamoyltransferase (GRMZM2G156816); CYP86A35, cytochrome P450 family 86, subfamily A, polypeptide 35 (GRMZM2G062151); UGT, UDP glycosyltransferases (GRMZM2G383404); WRKY53, superfamily of transcriptional factors having WRKY and zinc finger domains (GRMZM2G449681); RMVB, regulator of Vps4 activity in the MVB pathway protein (GRMZM2G059590); bx8, benzoxazinone synthesis 8 (GRMZM2G085054); ZFR, zinc finger, RING-CH-type (GRMZM2G358987); SDR, short-chain dehydrogenase/reductase (GRMZM2G000586); OXY, 2OG-Fe(II) oxygenase superfamily (GRMZM5G843555); PPR, PPR repeat domain containing protein (GRMZM2G325019). Full size image Naringenin is the key intermediate of the flavone/anthocyanin pathway, serving as the common precursor for a large number of downstream flavonoids, as described previously [46] . The occurrence of various flavones and O - or C -glycosyl flavones found here demonstrates the existence of the pathway including glycosyltransferase genes, implicating the genetic and biochemical basis for the formation of diverse flavonoids in the maize kernel. Metabolite GWAS thus facilitated characterization of the flavonoid metabolic pathway and identification of genes involved in its biosynthesis. Potential utilization of metabolites Reliable biomarkers significantly related to plant phenotypic performance is exceptionally attractive for breeders and plant biologists. Using variables with the highest significance above an arbitrary cutoff value, a set of candidate biomarkers can be defined [47] . In the present study, 26 metabolite features significantly associated with 100-kernel weight were detected in E2 that can explain 72.6% of the phenotypic variance. The most significant metabolite feature was n1043. For comparison, 17 significant metabolite features were found in E3, explaining 34.5% of the phenotypic variance. The most significant metabolite feature is n0486. Two metabolite features (that is, n0956 and n1618) were significant in both E2 and E3. It is demonstrated that a limited number of metabolite features significantly correlated with kernel weight ( P ≤0.05, general stepwise regression, N =335–339; Supplementary Table 3 ) can be explored as useful markers for plant breeding. Using 100-kernel weight as an example, five and two QTLs were found from linkage mapping in ZY and BB RIL populations, respectively. Forty-three QTLs of 42 metabolic traits identified in this study colocalized with these seven QTLs found for 100-kernel weight ( Supplementary Table 4 ). More interestingly, of these 42 metabolic traits, two (n1104 and n1266) were significantly associated with 100-kernel weight according to the general stepwise regression ( P ≤0.05; Supplementary Tables 3 and 4 ). Additionally, the strongest significant locus associated with n1266, which is also validated by linkage mapping, was exactly located in the region of a 100-kernel weight QTL identified in the ZY RIL population. Sixteen annotated genes were found within the ~500-Kb region including the lead candidate gene GRMZM2G066067 (annotated as a UDP-glucosyltransferase), and other genes such as GRMZM2G472651 (Thylakoid assembly4), GRMZM2G366373 (Aux/IAA-transcription factor), GRMZM2G141379 (Zinc finger, C3HC4 type), GRMZM2G112596 (ATPase-like), GRMZM2G043191 (Endonuclease/exonuclease/phosphatase), and so on ( Supplementary Fig. 11 ). Further evaluation and identification of the underlying genes will help to clone the QTL affecting the kernel weight as well as to understand the genetic architecture of complex traits, and thus further enhance the crop-breeding toolbox. Plants are rich in metabolites and it is critical to explore the immense diversity of plant metabolism for the products important to human well being [1] , [48] . Metabolites may exert control on growth either by acting as substrates for the synthesis of cellular components that become limiting under conditions of maximum growth, or by acting as signals regulating growth and development [13] , [49] . Many secondary metabolites are involved in biotic and abiotic stress responses. The economic value of maize grain and the very large contribution of maize to the diets of humans and animals make grain chemical composition studies an invaluable research target. The ability to understand quality determinants at the metabolic level, and use this information to boost grain nutrition, is one direct benefit of this study. By measuring 983 metabolite features that include 184 metabolites with associated chemical structures in kernels of 702 genotypes, our understanding of natural variation at the metabolite level of maize has largely furthered. More than 80% metabolite features identified in this study exhibited large fold change (>10) within maize lines, which suggested an interesting direction to explore how the huge quantitative variations regulate plant growth and development. GWAS has become a popular approach in plant genetic studies owing to the rapid advance of the sequencing technology in recent years [50] , [51] . Maize has exceptionally large diversity within species and rapid LD decay [51] . In our metabolite GWAS high analytical precision and marker density facilitated high-resolution mapping. We can achieve the mapping resolution down to a single gene in most cases in this study even though additional improvements will be possible with larger association panels as well as resolution and structure determination of a larger number of metabolites. Linkage mapping is an excellent tool for the validation of GWAS results. Rapidly developing genotyping platforms such as high-density SNP chip and genotyping by sequencing [52] will benefit the genotyping of larger panels of genotypes to achieve the identification of causative sequence variants. Availability of gene expression data owing to the RNA sequencing on our association panel also played an important role in validating function of candidate genes and investigating how the alleles work to change the phenotype. Picking and validating candidate genes would be significantly challenging in some cases based on current genomic annotation of maize. Function annotation of their orthologous genes in other species can be helpful clue to gain novel findings in maize, as shown by the cases of UGT and TDC in this study. Various approaches or tools are therefore useful and needed to interpret and utilize the GWAS results. Functional link between genetic variants and metabolic traits is relatively evident as suggested by our study, which demonstrates the great potential of combining genetics and metabolomics to dissect the biological mechanisms of maize metabolism. For instance, we updated the PAs and flavonoid biosynthetic pathways in this study. Our knowledge of both pathways is now greatly improved by the identification of previously unknown metabolites and candidate genes, including those for metabolic enzymes, transcription factor and transporters. Further studies, including structure confirmation of the selected metabolites and functional validation of additional candidate genes, can now be undertaken. Understanding natural variation at the metabolite level facilitates reconstruction of biosynthetic pathways, which in turn will benefit synthetic biology and metabolic engineering of desirable compounds in plants. Metabolites that are correlated with complex traits like biomass of plants possess great predictive power to be used as biomarkers [18] , [49] . A number of metabolite features significantly associated with kernel trait were identified in this study. Although further validation was required, the combination of GWAS and metabolomics provided an alternative to uncover agronomically important traits, which will enhance the molecular design breeding in maize as well as other crops. In summary, the combination of multiple technologies, including transcript and metabolite profiling, has facilitated candidate gene selection and allowed novel functional and biological insights into the association results. Future genetic studies in conjunction with genomics, transcriptomics, metabolomics and proteomics, as well as precision phenotyping, will help to fully uncover the mechanisms of complex agronomic and biochemical traits, and will lead to an accelerated rate of genetic gain in crop improvement. Populations and field trials Genetic materials used in this study included a panel of 368 diverse maize inbred lines for GWAS, which was referred to as the association panel [23] and two RIL populations, B73/By804 (ref. 53 ) and Zong3/Yu87-1 (ref. 54 ) for linkage analysis. Field trials for the association panel were conducted in three sites: Hainan (Sanya, E 109°51′, N 18°25′) in 2010, Yunnan (Kunming, E 102°30′, N 24°25′) and Chongqing (E 106°50′, N 29°25′) in 2011. These three experiments were hereafter referred to as E1, E2 and E3, respectively. The173 RIL lines from the B73/By804 cross (referred to as BB hereafter) were planted in Henan in 2011. The 161 RILs from the Zong3/Yu87-1 cross (referred to as ZY hereafter) were planted in Yunnan in 2011. All the inbred lines were divided into two groups (temperate and tropical/subtropical) based on pedigree information and planted in one-row plots in an incompletely randomized block design within the group. All lines were self-pollinated and ears of each plot were hand-harvested at their respective physiological maturity, followed by air drying and shelling. For each line, ears from five plants were harvested at the same maturity and bulked. One hundred kernels of each line were also counted and weighted for the association panel planted in three environments (Sichuan, 2009; Yunnan, 2009 and 2010) and for the two linkage populations planted in three environments (Chongqing, 2011; Hainan, 2011; Henan, 2011), respectively. The blup values of HKW across all environments were used for GWAS and linkage analysis. Genotyping and RNA sequencing All 368 lines of the association panel were genotyped using Illumina MaizeSNP50 BeadChip, which contains 56,110 SNP loci [55] . Ninety-base pair pair-end Illumina RNA sequencing was subsequently performed on the immature seeds of 15 days after pollination for these 368 lines. In all, 1.06 million high-quality SNPs were identified in the whole panel and the expression data for 28,769 genes were also obtained in all the 368 lines. The detailed information was described in the recent studies [22] , [23] . Both RIL populations have been genotyped using Illumina GoldenGate BeadChip containing 1,536 SNPs and linkage map was constructed for both populations [56] . Sample preparation and metabolite profiling We carried out metabolic profiling on mature maize kernels from lines of the association panel ( n =368) and two RIL populations ( N =173 and 167, respectively). For each line, 12-well growth kernels were randomly selected from five plants and bulked for grinding. The kernels were ground using a mixer mill (MM 400, Retsch) with zirconia beads for 2.0 min at 30 Hz. The powder of each genotype was partitioned into two sample sets and stored at −80 °C until they were required for extraction. One sample set was extracted for lipid-soluble metabolites, while the other was for extracting water-soluble metabolites. One hundred milligram of powder and 1 ml absolute methanol, which contained 0.1 mg l Lincomycin and Lidocaine, were used for lipid-soluble metabolites (or 70% methanol for water-soluble metabolites). Samples were extracted overnight at 4 °C. After centrifugation at 10,000 g for 10 min, 0.4 ml of each extract was combined and filter spun using 0.22-μm filters (ANPEL, Shanghai, China, http://www.anpel.com.cn/ ) before analysis using an LC-ESI-MS/MS system. The metabolite quantification and annotation is performed by our newly developed method [57] , which is described in detail in the Supplementary Notes . All the data are reported in detail in the Supplementary Materials , following the recommendations for reporting metabolite data by Fernie et al . [58] (see the Supplementary Note 1 ; Supplementary Data 1 and 2 and Supplementary Fig. 12 ). Metabolite identification and annotation To facilitate the identification/annotation of detected metabolites by our widely targeted metabolomics approach, accurate m / z of each Q1 was obtained, if possible. To this end, extracted ion chromatograms (XICs) of the ESI-QqTOF-MS data for each of Q1 ( m / z ±0.2 Da) of the 983 transitions in the MS2T library were manually evaluated for the presence of the targeted substances by analysing corresponding mass spectra, and the accurate m / z values were obtained. For each of the corresponding accurate m / z , fragmentation pattern was obtained by running the analysis under targeted MS/MS mode using three different collision energies of 10, 20 and 30 eV. The accurate m / z was assigned to the corresponding Q1 if similar fragmentation patterns were obtained between the ESI-Q TRAP-MS/MS and the ESI-QqTOF-MS/MS. Eventually, accurate mass of 245 of Q1 was obtained. The MS2T library was annotated based on the fragmentation pattern (delivered by ESI-Q TRAP-MS/MS and/or the accurate m / z value delivered by ESI-QqTOF-MS/MS) and the retention time of each metabolite. Based on the annotation, commercially available standards were purchased and analysed using the same profiling procedure as the extracts. By comparing the m / z values, the retention time and the fragmentation patterns with the standards, 49 metabolites were identified, including amino acids, flavonoids, lysoPCs and fatty acid (such as α-linolenic acid), and some phytohormones (see Supplementary Data 2 ). For the metabolites that couldn’t be identified by available standards, peaks in the MS2T library, especially the peaks that have similar fragmentation patterns with the metabolites identified by authentic standards, were used to query the MS/MS spectral data taken from the literature or to search the databases (MassBank, KNApSAcK, HMDB, MoTo DB and METLIN). Best matches were then searched in the Dictionary of Natural products and KEGG for possible structures. In all, 184 metabolites were identified and more than four different pathways were detected in our study. Statistical analysis of metabolic traits The mixture of 150 randomly chosen extracts from the association panel was used as a reference control of each measured batch [59] . One reference control that contains 983 molecular features was placed and measured per 25 genotypes. In our study, the reference control were used for normalization even though two internal standards were added, since we think the internal standards are not the best to reflect the change of all metabolite features through the analysis procedure, considering different properties of the large number of metabolite features we analysed. Moreover, each set of 25 samples and each molecular feature were normalized to the average level of reference control that was injected before and after these 25 samples. All procedures were applied after normalization of the metabolite data using the reference control. All the metabolite concentrations were log 2 -transformed for further analysis. Since only one replication was performed in each experiment, phenotypic variance ( V p ) was partitioned into genotype ( V g ), environment ( V e ) and the error ( V er ) using a SAS proc mixed procedure. Repeatability ( R ) was then calculated for each metabolite as R = V g / V p according to Holland et al. [60] Genome-wide association studies Given that the MS system for E1 was different from that used in the other two experiments ( Supplementary Note 1 ), for simplicity, GWAS was independently performed for each metabolic trait obtained in each experiment. We used a compressed mixed linear model [61] accounting for the population structure ( Q ) and familial relationship ( K ) [23] to examine the association between SNPs and metabolic traits. SNPs with a moderate minor allele frequency (MAF>5%) in the 368 lines were employed in the association analysis. P value of each SNP was calculated and significance was defined at a uniform threshold of ≤1.8 × 10 −6 ( P =1/ n ; n =total markers used, which is roughly a Bonferroni correction). SNP with the lowest P value (that is, lead SNP) and its corresponding gene were reported for each significant metabolic locus (see Supplementary Data 3 ). To validate each significant locus by linkage analysis, the physical position of its lead SNP was compared with the physical region of QTL. For the purpose of evaluating each candidate gene, eQTL analysis was conducted to investigate the regulatory pattern of each gene, and the relationship between its expression level and the corresponding metabolic trait was further investigated. Linkage mapping We conducted QTL analysis using Composite Interval Mapping implemented in Windows QTL Cartographer V2.5 (refs 62 , 63 ) for metabolites detected in the two RIL populations. Zmap (model 6) with a 10-cM window and an interval-mapping increment of 2 cM were used. To determine a uniform threshold for significant QTLs 1,000 permutations were used for 100 randomly selected traits, 50 traits from each RIL population. The average LOD value at P <0.05 is 2.88, so we chose a uniform value (LOD=3) as the cutoff. The genomic region in which a peak of LOD value reached the threshold (LOD=3), and the LOD of the flanking markers was >2.5, was designated as a confidence interval. eQTL mapping Using the same method as for GWAS, the associations between genome-wide SNPs and the expression level of each metabolic trait-associated gene were investigated. SNPs within a 100-kb region of the lead SNP for each metabolic trait were evaluated for their possible regulatory involvement. Only genes expressed in >50% of the 368 sequenced lines that had a mean quantification of >10 reads were used in this analysis. Vector construction and rice transformation The over-expression vector (pJC034) for rice is constructed from the gateway over-expression vector pH2GW7; 35S promoter of pH2GW7 is replaced by maize ubiquitin promoter, which is more suitable for rice over-expression study. To generate PHT and CCoAOMT1 over-expression constructs, the full-length cDNA of PHT was amplified from maize inbred line B73 by reverse transcription (RT)-PCR. The PCR product was cloned into the gateway vector pDONR207 using the BP enzyme (Invitrogen, Shanghai, China), and then sequenced; the right clones would be used for LR reaction with pJC034 using the LR enzyme (Invitrogen, Shanghai, China). This construct were introduced into japonica rice cultivar ZH11 by Agrobacterium tumefaciens -mediated transformation [64] . Expression analyses of the transformed genes We isolated total RNA from rice and maize leaves using an RNA extraction kit (TRIzol reagent; Invitrogen, Shanghai, China) according to the manufacturer’s instructions. The first-strand cDNA was synthesized using MLV (Invitrogen, Shanghai, China) according to the manufacturer’s protocol. Real-time PCR was performed on an optical 96-well plate in an ABI SteponePlus PCR system (Applied Biosystems, Shanghai, China) by using SYBR Premix reagent F-415 (Thermo scientific, Shanghai, China). The relative expression level of gene PHT and CCoAOMT1 was determined with the rice Actin1 (ref. 65 ) gene as an internal control. The expression measurements were obtained using the relative quantification method [66] . For semi-quantitative RT-PCR, reactions were performed in 20-μl volumes with the following protocol: one cycle of 94 °C for 5 min and 30 cycles of 94 °C for 30 s, 58 °C for 30 s and 72 °C for 60 s. Detection of metabolites significantly associated with 100-kernel weight General step-wise regression, implemented by GLMSelect procedure in SAS software [67] , was used to detect metabolites significantly associated with 100-kernel weight investigated in E2 and E3. The probability of marker entering into the model was set at 0.05 for selecting the top metabolites. Data availability All data are available as a public resource to aid functional studies and interpretation of GWAS findings. Data sets including genotypic, phenotypic, expression and the mass spec data of each line and detailed information of called SNPs from RNA-sequencing result can be viewed and downloaded from the website http://www.maizego.org/Resources.html . Accession Codes : RNA sequencing data of 368 maize inbred lines have been deposited in the GenBank Sequence Read Archive (SRA) under the accession code SRP026161 . How to cite this article: Wen, W. et al. Metabolome-based genome-wide association study of maize kernel leads to novel biochemical insights. Nat. Commun. 5:3438 doi: 10.1038/ncomms4438 (2014).